Benzene- and pyridine-incorporated octaphyrins with different coordination modes toward two PdIIcenters Expanded porphyrins have received considerable attention due to their unique optical, electrochemical and coordination properties. Here, we report benzene- and pyridine-incorporated octaphyrins(1.1.0.0.1.1.0.0), which are synthesized through Suzuki-Miyaura coupling of α,α′-diboryltripyrrane with m- dibromobenzene and 2,6-dibromopyridine, respectively, and subsequent oxidation with 2,3-dicyano-5,6-dichlorobenzoquinone. Both octaphyrins are nonaromatic and take on dumbbell structures. Upon treatment with Pd(OOCCH 3 ) 2 , the benzene-incorporated one gives a C i symmetric NNNC coordinated bis-Pd II complex but the pyridine incorporated one gives C i and C s symmetric NNNC coordinated bis-Pd II complexes along with an NNNN coordinated bis-Pd II complex bearing a transannular C–C bond between the pyrrole α-positions. In addition, these two pyridine-containing NNNC Pd II complexes undergo trifluoroacetic acid-induced clean interconversion. In recent years, considerable attention has been focused on expanded porphyrins in light of their attractive optical, electrochemical, and coordination properties [1] , [2] , [3] , [4] , [5] , [6] , [7] , [8] , [9] , [10] , [11] , [12] . Among these, pyridine-incorporated expanded porphyrins possess a unique position, since they showed interesting chemical behaviors arising from the basic pyridine subunits. More than two decades ago Corriu et al. reported the synthesis of benzene-incorporated and pyridine-incorporated amethyrin analogs 1 and 2 via a rational route [13] . Later, several analogous molecules possessing unique functions have been reported. As representative examples, cryptand-like molecule 3 exhibited unique properties such as binding three ethanol molecules and positive cooperativity in binding carboxylic acids [14] . Cyclo[2]pyridine[4]pyrrole 4 and cyclo[3]pyridine[3]pyrrole 5 showed protonation-induced realization of global conjugated networks [15] and supramolecular assembling with dicarboxylic acids [16] . Pyridine-modified rubyrin 6 underwent protonation-induced flipping of the pyridine subunits [17] , and cyclo[6]pyridine[6]pyrrole 7 was synthesized as the largest pyridine-incorporating expanded porphyrin that showed characteristic conformational flexibility (Fig. 1 ) [14] , [15] , [16] , [17] , [18] , [19] , [20] , [21] , [22] , [23] . Fig. 1: Representative structures of benzene-incorporated or pyridine-incorporated expanded porphyrinoids 1 – 8 . 1 , benzene-incorporated amethyrin analog; 2 , pyridine-incorporated amethyrin analog; 3 , cryptand-like molecule; 4 , cyclo[2]pyridine[4]pyrrole; 5 , cyclo[3]pyridine[3]pyrrole; 6 , pyridine-modified rubyrin; 7 , cyclo[6]pyridine[6]pyrrole; 8 , octaphyrin. Full size image Recently we explored various porphyrinoids by using Suzuki–Miyaura coupling. Reported examples include cyclic porphyrin rings, BODIPY-porphyrin hybrids, and earring porphyrins [24] , [25] , [26] , [27] , [28] . Despite of these studies, we thought that this coupling strategy could be applied to the synthesis of pyridine-incorporated expanded porphyrins. [36]Octaphyrins(1.1.1.1.1.1.1.1) 8 have been known to bind two metal ions within two semi-porphyrin-like pockets and their bis-Cu II and bis-Co II complexes were demonstrated to undergo quantitative splitting reactions to give the corresponding two metaloporphyrins almost quantitatively [29] , [30] . Here, we report the synthesis of phenylene-incorporated and pyridine-incorporated octaphyrins that have remained largely unexplored. The presence of pyridine units into the octaphyrin scaffold leads to unexpected metalation modes and reactivity of the resultant metal complexes. Since the pyridine is quite basic it enables preferential protonation and metal coordination. The pyridine-incorporated octaphyrin coordinates Pd II to form C i and C s symmetric NNNC bis-Pd II complexes, and an NNNN coordinated bis-Pd II complex bearing a transannular C–C bond between the pyrrole α-positions. The former two complexes can interconvert upon addition of trifluoroacetic acid (TFA). Synthesis and structural characterization of 12 and 14 1,3-Phenylene-incorporated and 2,6-pyridylene-incorporated octaphyrins(1.1.0.0.1.1.0.0) 12 and 13 are the target molecules in the present study. The key precursor α,α′-Diboryltripyrrane 9 was prepared by regioselective Ir-catalyzed borylation of 5,10-dimesityltripyrrane (Fig. 2 ) [28] . Firstly, we tried the synthesis of 1,3-phenylene-incorporating octaphyrin 12 by Suzuki-Miyaura coupling of 9 with m- dibromobenzene and subsequent oxidation with 2,3-dichloro-5,6-dicyano-1,4-benzoquinone (DDQ) but this reaction sequence gave linear precursor 10 in 53% yield. We then examined the cyclization of 10 with 9 under similar coupling and oxidation conditions. The equimolecular reaction of 9 and 10 yielded 12 in 3.8% yield but the yield of 12 could be improved to 8.0% when 1.2 equivalent of 9 was applied. The parent ion peak of 12 was detected at m / z = 1062.5479 (calcd for [C 76 H 66 N 6 ] + = 1062.5343 [M] + ). The 1 H nuclear magnetic resonance (NMR) spectrum shows a symmetric feature displaying a broad singlet at 13.00 ppm due to the pyrrolic NH protons, two doublets at 7.39 and 7.03 ppm and a singlet at 6.33 ppm due to the pyrrolic β-protons, and only three singlet signals due to the methyl protons of the mesityl groups. Collectively, these chemical shifts indicate a nonaromatic character for 12 (see Supplementary Fig. 4 and Supplementary Table 8 ). Fortunately, we obtained single crystals of 12 by slow diffusion of isopropanol vapor into its chlorobenzene solution. As shown in Fig. 3a, b , 12 takes a planar dumbbell structure with C i symmetry, in which the two 1,3-phenylene units are pointing inward, being close to overlapping, and the two tripyrrin units are also pointing inward, forming two hemiporphyrin-like pockets. There is no particular bond-length alteration in the 1,3-phenylene units. Fig. 2: Syntheses of 12-17 . Reaction conditions: i) excess m- dibromobenzene or 2,6-dibromopyridine, Pd 2 (dba) 3 , PPh 3 , Cs 2 CO 3 , CsF, p- xylene or toluene/DMF, reflux, 48 h. ii) DDQ, CH 2 Cl 2 , r.t. iii) α,α′-diboryltripyrrane Pd 2 (dba) 3 , PPh 3 , Cs 2 CO 3 , CsF, p- xylene or toluene/DMF, reflux, 48 h. iv) DDQ, CH 2 Cl 2 , r.t. v) m- dibromobenzene or 2,6-dibromopyridine, Pd 2 (dba) 3 , PPh 3 or XPhos, Cs 2 CO 3 , CsF, toluene/DMF, reflux, 48 h. vi) DDQ, CH 2 Cl 2 , r.t. vii) Pd(OAc) 2 , NaOAc, CHCl 3 /CH 3 OH, reflux. dba = dibenzylideneacetone, Mes = 2,4,6-trimethylphenyl, Bpin = pinacolatoboryl. Full size image Fig. 3: X-ray structures of 12 and 14 . a Top view and b side view of 12 . c top view, and d side view of 14 . The thermal ellipsoids are on 30% probability level. Hydrogen atoms except those connected to N atoms are omitted for clarity. Carbon atom, black ellipsoid; nitrogen atom, blue; palladium atom, orange; hydrogen atom small black ball. Full size image Encouraged by the hemiporphyrin-like pockets, we examined Pd II metalation of 12 . A solution containing 12 , Pd(OAc) 2 , and NaOAc in a mixture of chloroform and methanol was refluxed for 24 h, which yielded 14 in 74% yield as a single product. The parent ion peak was detected at m / z = 1270.3018 (calcd for [C 76 H 62 N 6 Pd 2 ] + = 1270.3134 [M] + ). The structure of 14 was also determined by single crystal X-ray diffraction analysis (Fig. 3c,d ). Complex 14 shows a C i structure, in which the two Pd II ions take square planar coordination bound with the three pyrrolic nitrogen atoms and one carbon atom in the 1,3-phenylene unit. Synthesis and structural characterization of 13 , 15 , 16, and 17 By following the stepwise synthetic protocol for 10 , α,α′-di(6-bromopyrid-2-yl)tripyrrin 11 was prepared by the reaction of 9 with 2,6-dibromopyridine in 48% yield, and octaphyrin 13 was synthesized by the reaction of 9 with 11 in 9.0% yield. The direct one-pot method gave 13 in 8.1% yield. The parent ion peak of 13 was observed at m / z = 1064.5239 (calcd for [C 74 H 64 N 8 ] + 1064.5248 [M] + ) and the 1 H NMR spectrum of 13 is similar to that of 12 , indicating its symmetric structure and a nonaromatic character. Octaphyrin 13 shows a planar dumbbell structure quite similar to that of 12 , in which the two hemiporphyrin-like cavities are secured (Fig. 4a, b ). Fig. 4: X-ray structures of 13 , 15, and 16 . a Top view. b Side view of 13 . c Top view and d) side view of 15 . e Top view and f side view of 16 . The thermal ellipsoids are on 30% probability level. Hydrogen atoms are omitted for clarity. Carbon atom, black ellipsoid; nitrogen atom, blue; palladium atom, orange; hydrogen atom small black ball. Full size image Considering the high coordination ability of pyridine, it was thought that metalation behaviors of 13 might be different from those of 12 . Pd II metalation of 13 under the same conditions afforded three Pd II complexes 15 , 16 , and 17 in 20%, 60%, and 12% yield, respectively. The structures of 15 and 16 are analogous to that of 14 but that of 17 is substantially different. The parent ion peaks of 15 and 16 were observed at m / z = 1272.2944 (calcd for [C 74 H 60 N 8 Pd 2 ] + 1272.3038 [M] + ) and m / z = 1272.3063 (calcd for [C 74 H 60 N 8 Pd 2 ] + 1272.3038 [M] + ), respectively. Structures of 15 and 16 were unambiguously determined by X-ray analysis as shown in Fig. 4c–f . Both complexes show the similar planar dumbbell structures but differ in Pd II coordination modes. Namely, in 15 the Pd II metals are respectively bound to different pyridine units, while the two Pd II metals in 16 are bound to the same pyridine unit in a C s symmetric manner. The Pd–N bond lengths are 1.969(5), 1.978(6), 2.053(6), 2.069(6), 2.071(5), and 2.085(6) Å, and Pd–C bond lengths are 2.077(7) and 2.102(7) Å in 16 . The sum of the bond angles around the Pd ions are 361.4(3)° and 361.1(3)° for 16 , being closer to the ideal square-planar coordination geometry. In line with these structures, the 1 H NMR spectrum of 15 shows a set of doublets at 5.46 and 4.07 ppm due to the 2,6-pyridinylene units and that of 16 displays a singlet at 3.69 ppm and a set of mutually coupled doublet at 7.67 ppm and a triplet at 7.03 ppm. These chemical shifts can be explained by the local aromaticity of 1,3-phenylene and 2,6-pyridylene, which meet well with the NICS calculation. DFT calculation reveals that either in 15 or 16 d orbitals of Pd atoms are clearly involved in the HOMO and LUMO orbitals, which indicates a strong electron interaction between Pd atoms and octaphyrin scaffolds. The structure of 17 is shown in Fig. 5 . The Pd1 atom is coordinated with three pyrroles B, C, D and pyridine A in a square planar manner with bond lengths of 1.922(3), 1.962(6), 1.942(4), and 2.024(5) Å. The Pd2 atom is bounded to the three nitrogen atoms of pyrrole rings F, G, H and pyridine E with distances of 1.926(4), 1.971(5), 1.947(4), and 2.023(4) Å. This hemi-porphyrin-like unit is relatively planar with a small mean plane deviation of 0.037(6) Å. Surprisingly, a new C–C bond is formed between the α-positions of the pyrroles D and H, causing a disruption of the macrocyclic conjugated network. This transannular bond length is rather large, being 1.568(8) Å. As a consequence, complex 17 exhibits a roughly perpendicular arrangement of two hemiporphyrin-like units. The parent ion peak was detected at m / z = 1274.3141 (calcd for [C 74 H 62 N 8 Pd 2 ] + 1274.3195 [M] + ), which is two units larger than those of 15 and 16 . The 1 H NMR and 13 C NMR spectra are consistent with the structure. Characteristically, the 13 C NMR spectrum shows a signal at 91.44 ppm due to the sp 3 -hybridized quaternary carbon atoms. The detailed reaction mechanism is not clear but may involve the bis-Pd II complex 18 , which may be highly distorted and undergo a transannular C–C bond forming reaction to give 17 (Fig. 6 ). This process differs from the previous transannular reactions of expanded porphyrins (Fig. 7 ) [30] , [31] , [32] , [33] , [34] , [35] . Fig. 5: X-ray structure: 17 . The thermal ellipsoids are on 30% probability level. Hydrogen atoms except those in 2,6-pyridylene are omitted for clarity. Carbon atom, black ellipsoid; nitrogen atom, blue; palladium atom, orange; hydrogen atom small black ball. Full size image Fig. 6: Plausible reaction mechanism from 13 to 17 . 13 to 13′ , conformation variation via σ bond rotation; 13′ to 18 , metal coordination; 18 to 17 , C–C bond (red) forming. Full size image Fig. 7: Absorption spectra of 12–17 in CH 2 Cl 2 . UV–Vis–NIR absorption spectra of 12 (blue), 14 (green), 13 (purple), 15 (black), 16 (red), and 17 (khaki). λ , wavelength; ε molar extinction coefficient. 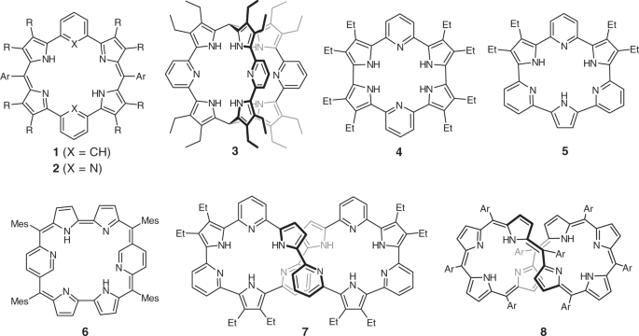Fig. 1: Representative structures of benzene-incorporated or pyridine-incorporated expanded porphyrinoids1–8. 1, benzene-incorporated amethyrin analog;2, pyridine-incorporated amethyrin analog;3, cryptand-like molecule;4, cyclo[2]pyridine[4]pyrrole;5, cyclo[3]pyridine[3]pyrrole;6, pyridine-modified rubyrin;7, cyclo[6]pyridine[6]pyrrole;8, octaphyrin. Full size image Electrochemical and optical properties of 12, 13, 14, 15, 16, and 17 Cyclic voltammetry (CV) and differential-pulse voltammetry (DPV) experiments were conducted and the redox potentials are summarized in Table 1 . Table 1 Electrochemical properties of 12 , 14 , 13 , 15 , 16 , and 17 measured in PhCN. Full size table In all cases, the oxidation waves are irreversible, indicating certain instabilities under oxidative conditions. On the other hands, the first and second reduction waves are reversible, showing a stepwise 1e – reduction at –1.31 and –1.48 V for 12 , at –1.07 and –1.29 V for 14 . The Pd II complexation result in a definitive anodic shift by about 0.2 V. It is also the case for 13 , the reduction peaks were observed at –0.92 and –1.18 V for 15 and at –0.97 and –1.20 V for 16 , both of which were anodically shifted from those of 13 . Interestingly, the first oxidation potential of 16 (0.47 V) is more negatively shifted than that of 15 (0.62 V), resulting in the smallest gap (Δ E HL ) of 1.44 eV. The Δ E HL values of 14 and 15 are almost identical, which is consistent with the orders of absorption red-shifts. The first oxidation potential of 17 was observed at –0.02 V, indicating its electron rich nature. This may be accounted for the presence of two 2-hydropyrrole units in 17 . The UV-Vis absorption spectra of 12 and 13 are quite similar, exhibiting bands at 402, 551, and 598 nm and at 406, 555, and 610 nm, respectively. The absorption spectrum of 14 is broader and red-shifted, showing bands at 422, 599, and 700 nm. 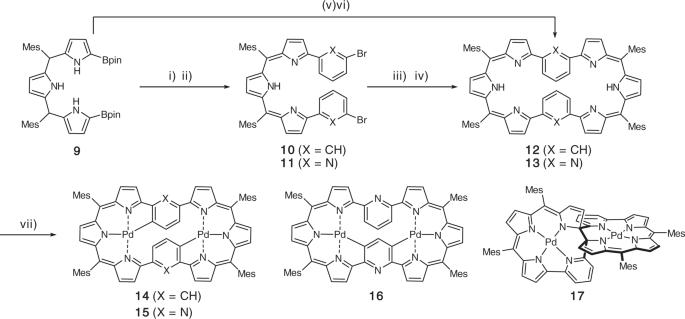Fig. 2: Syntheses of12-17. Reaction conditions: i) excessm-dibromobenzene or 2,6-dibromopyridine, Pd2(dba)3, PPh3, Cs2CO3, CsF,p-xylene or toluene/DMF, reflux, 48 h. ii) DDQ, CH2Cl2, r.t. iii) α,α′-diboryltripyrrane Pd2(dba)3, PPh3, Cs2CO3, CsF,p-xylene or toluene/DMF, reflux, 48 h. iv) DDQ, CH2Cl2, r.t. v)m-dibromobenzene or 2,6-dibromopyridine, Pd2(dba)3, PPh3or XPhos, Cs2CO3, CsF, toluene/DMF, reflux, 48 h. vi) DDQ, CH2Cl2, r.t. vii) Pd(OAc)2, NaOAc, CHCl3/CH3OH, reflux. dba = dibenzylideneacetone, Mes = 2,4,6-trimethylphenyl, Bpin = pinacolatoboryl. The absorption spectra of 15 and 16 are even broader and red-shifted. The spectral profiles of 15 and 16 are similar in the range of 350–500 nm but are different in the low energy region. Namely, 15 shows a tail up to 850 nm but 16 shows a tail reaching around 1000 nm. The absorption spectrum of 17 is also broader and red-shifted, exhibiting absorption bands at 444, 651, and 697 nm. Upon addition of acid, the absorption spectrum of 13 was largely changed probably due to the protonation of the pyridine moieties, since the addition of acid to CH 2 Cl 2 solution of 12 did not lead to any changes in its UV–Vis spectrum (Supplementary Fig. 27 ). Mutual interconversion between 15 and 16 In the meanwhile, we found TFA-triggered clean mutual interconversion between 15 and 16 . In neutral or basic solutions, the mutual interconversion was not detected even at high temperature. Small amounts of TFA (0.05 or 0.2 equiv) accelerated the interconversion with molar ratios of 15 / 16 at the saturation point: 3.2 or 1.1 (see Supplementary Figs. 40 and 41 ). On the other hand, in the presence of 1.0 or 2.0 equiv TFA, the interconversion was rapid but gave 16 predominantly (see Supplementary Figs. 42 and 43 ). After certain reaction time, the interconversion showed the same saturation feature starting from either 15 or 16 , suggesting thermodynamic control. We thought that the relative stability of neutral 15 to 16 determined the equilibrium at low concentration of TFA and that of monoprotonated 15 to 16 determined the equilibrium at high concentration of TFA. TFA-d was then applied to explore the process of proton transferring process. Spectra of the product 16-d indicated that C–H activation and the following C–Pd bonds deuteration underwent in the isomerization process. To better understand this process DFT calculations of the relative energies of 15 and 16 in neutral and monoprotonated forms were conducted (see Supplementary Figs. 56 and 57 ). In the monoprotonated forms, the most stable form was 16 protonated at the Pd-coordinated pyridine site, which is 9.0 kcal/mol more stable than 15 , in line with the experimental results. In contrast, the Gibbs free energy difference between neutral 15 and 16 is subtle (~2.7 kcal/mol), so that the equilibrium may be influenced by solvent effects or other experimental conditions. In summary, the benzene and pyridine incorporating octaphyrins 12 and 13 were synthesized through Suzuki–Miyaura coupling reaction of the simple starting materials and subsequent oxidation with DDQ. These octaphyrins are nonaromatic and show dumbbell structures. The incorporation of pyridine units into the octaphyrin framework has strong influences such as the formation of the isomeric bis-Pd II complexes 15 and 16 along with the rearranged complex 17 . Further, the complexes 15 and 16 underwent the TFA-induced mutual interconversion depending upon the concentration of TFA. Further exploration of core-modified expanded porphyrins is underway in our laboratories. Materials, characterizations, and theoretical calculations 1 H NMR (500 MHz) spectra were measured by a Bruker AVANCE-500 spectrometer, and chemical shifts were reported on the delta scale in ppm relative to CHCl 3 as an internal reference ( δ = 7.260 ppm). Assignments of 1 H NMR were based on HH COSY spectra and D 2 O exchange experiments. UV/Vis absorption spectra were recorded on a Shimadzu UV-3600 spectrometer. X-ray crystallographic data were taken on an Agilent SuperNova X-ray diffractometer equipped with a large area CCD detector. Using Olex2, structures of compounds 12 – 17 were solved with the ShelXS structure solution program using Direct Methods and refined with the ShelXL refinement package using Least Squares minimization. Disordered solvent molecules were treated by SQUEEZE program of Platon. Redox potentials were measured by the cyclic voltammetry and differential pulse voltammetry method on an ALS660 electrochemical analyzed model (Solvent: PhCN, electrolyte: 0.1 M n-Bu 4 NPF 6 , working electrode: glassy carbon, reference electrode: Ag/AgNO 3 , Counter electrode: Pt wire, scan rate: 0.05 V/s, external reference: ferrocene/ferrocenium cation). Benzonitrile passed through alumina column was used for electrochemical analysis. Unless otherwise noted, materials obtained from commercial suppliers were used without further purification. All calculations were carried out using the Gaussian 09 program [36] . Initial geometries for 12–17 were obtained from X-ray structures. The structures were fully optimized without any symmetry restriction. Geometry optimizations in the ground state ( S 0 ) were performed by the density functional theory (DFT) method with restricted B3LYP (Becke’s three-parameter hybrid exchange functionals and the Lee–Yang–Parr correlation functional) [37] , [38] level employing basis sets and pseudopotentials; 6–311G(d,p) for C, H, N [39] , and SDD for Pd [40] . NICS(0) values were calculated with GIAO method at the B3LYP level employing the same basis sets and pseudopotentials for geometry optimizations. Calculated chemical shifts were estimated relative to the magnetic shielding of a proton of chloroform (24.95 ppm) calculated at the same level. Synthesis of 10 A toluene-DMF solution (3/1.5 mL) of 9 (178.4 mg, 0.25 mmol), 1,3-dibromobenzene (301.7 μL, 589.8 mg, 2.5 mmol), Pd 2 (dba) 3 (22.9 mg, 0.025 mmol), PPh 3 (26.2 mg, 0.1 mmol), Cs 2 CO 3 (172.7 mg, 0.53 mmol), and CsF (77.5 mg, 0.51 mmol) was degassed through three freeze-pump - thaw cycles, and the reaction Schlenk tube was purged with argon. The resulting mixture was stirred at reflux for 48 h. The reaction mixture was diluted with CHCl 3 , washed with water, and dried over anhydrous sodium sulfate. After the solvent was removed, 2,3-dichloro-5,6-dicyano-1,4-benzoquinone (DDQ) (136.2 mg, 0.6 mmol) was added to the resulting mixture in CH 2 Cl 2 and this reaction mixture was stirred for another 4 h. Evaporation of the solvent followed by silica-gel column chromatography (CH 2 Cl 2 /n-hexane as an eluent) and recrystallization with CH 3 OH to afford 10 as dark green solids (101.7 mg, 0.13 mmol, 53% yield). 1 H NMR (500 MHz) (CDCl 3 ) δ = 13.60 (br, 1H), 8.00 (s, 2H), 7.68 (d, 2H, J = 7.7 Hz), 7.20 (d, 2H, J = 8.0 Hz), 7.14 (d, 2H, J = 4.5 Hz), 6.97 (s, 4H), 6.88 (d, 2H, J = 4.5 Hz), 6.75 (t, 2H, J = 7.6 Hz), 6.19 (s, 2H), 2.38 (s, 6H), 2.18 (s, 12H) ppm; 13 C NMR (126 MHz) (CDCl 3 ): δ = 168.2, 152.7, 139.0, 137.7, 137.3, 137.0, 135.7, 133.6, 132.1, 131.0, 128.8, 127.9, 126.8, 124.1, 122.1, 121.0, 21.1, and 20.5 ppm; HRMS ( m / z ): [M] + calcd. for C 44 H 37 Br 2 N 3 , 765.1349; found 765.1291. Synthesis of 11 A toluene-DMF solution (3/1.5 mL) of 9 (178.4 mg, 0.25 mmol), 2,6-dibromopyridine (592.2 mg, 2.5 mmol), Pd 2 (dba) 3 (22.9 mg, 0.025 mmol), PPh 3 (26.2 mg, 0.1 mmol), Cs 2 CO 3 (172.7 mg, 0.53 mmol), and CsF (77.5 mg, 0.51 mmol) was degassed through three freeze-pump-thaw cycles, and the reaction Schlenk tube was purged with argon. The resulting mixture was stirred at reflux for 48 h. The reaction mixture was diluted with CHCl 3 , washed with water, and dried over anhydrous sodium sulfate. After the solvent was removed, DDQ (136.2 mg, 0.6 mmol) was added to the resulting mixture in CH 2 Cl 2 and this reaction mixture was stirred for another 4 h. The reaction mixture was passed through a short alumina column (CH 2 Cl 2 as an eluent) and recrystallization with CH 3 OH to afford 11 as dark green solids (91.9 mg, 0.119 mmol, 47.8% yield). 1 H NMR (500 MHz) (CDCl 3 ): δ = 13.31 (br, 1H), 7.47 (m, 4H), 7.27 (d, 2H), 6.97 (s, 4H), 6.89 (d, 2H, J = 4.5 Hz), 6.66 (t, 2H, J = 7.6 Hz), 6.28 (s, 2H), 2.38 (s, 6H), 2.16 (s, 12H) ppm. 13 C NMR (126 MHz) (CDCl 3 ): δ = 168.4, 153.2, 153.0, 140.8, 139.4, 139.0, 138.0, 137.5, 137.1, 135.5, 133.4, 128.0, 127.5, 125.9, 121.9, 121.8, 21.1, 20.5 ppm; HRMS ( m / z ): [M+H] + calcd. for C 42 H 36 Br 2 N 5 , 768.1332; found 768.1354. Synthesis of 12 Route 1: A p- xylene-DMF solution (3/1.5 mL) of 9 (84 mg, 0.12 mmol), 10 (77.7 mg, 0.1 mmol), Pd 2 (dba) 3 (18.5 mg, 0.02 mmol), PPh 3 (21.2 mg, 0.08 mmol), Cs 2 CO 3 (71.0 mg, 0.2 mmol), and CsF (33.4 mg, 0.2 mmol) was degassed through three freeze-pump-thaw cycles, and the reaction Schlenk tube was purged with argon. The resulting mixture was stirred at reflux for 48 h. The reaction mixture was diluted with CHCl 3 , washed with water, and dried over anhydrous sodium sulfate. After the solvent was removed, DDQ (65.8 mg, 0.29 mmol) was added to the resulting mixture in CH 2 Cl 2 , and this reaction mixture was stirred for another 8 h. The reaction mixture was passed through a short alumina column (CH 2 Cl 2 as an eluent). Evaporation of the solvent followed by silica-gel column chromatography (CH 2 Cl 2 /n-hexane as an eluent) and recrystallization with CH 2 Cl 2 /MeOH afforded 12 as violet solids (8.4 mg, 0.008 mmol, 8.0% yield). Route 2: A toluene-DMF solution (3/1.5 mL) of 9 (180 mg, 0.25 mmol), 1,3-dibromobenzene (25.6 μL, 49.5 mg, 0.21 mmol), Pd 2 (dba) 3 (23 mg, 0.025 mmol), X-Phos (48 mg, 0.10 mmol), Cs 2 CO 3 (136.0 mg, 0.42 mmol), and CsF (67.0 mg, 0.44 mmol) was degassed through three freeze-pump-thaw cycles, and the reaction flask was purged with argon. The resulting mixture was stirred for 48 h at reflux. The reaction mixture was diluted with CHCl 3 , washed with water, and dried over anhydrous sodium sulfate. After the solvent was removed, DDQ (136.2 mg, 0.6 mmol) was added to the resulting mixture in CH 2 Cl 2 and this reaction mixture was stirred for another 8 h. The reaction mixture was passed through a short alumina column (CH 2 Cl 2 as an eluent). Evaporation of the solvent followed by column chromatography on silica gel (CH 2 Cl 2 /n-hexane as an eluent) and recrystallization from n-hexane gave 12 as violet solids (7.9 mg, 0.007 mmol, 7.0% yield) 1 H NMR (500 MHz) (CDCl 3 ): δ = 13.0 (br, 2H, N–H), 8.34 (br, 2H, m- phenylene-H), 7.39 (d, 4H, J = 4.5 Hz, pyrrole-H), 7.25 (dd, 4H, J = 7.8, 1.5 Hz, m- phenylene-H), 7.03–7.00 (m, 12H, pyrrole-H and Ar- m- H), 6.33 (s, 4H, pyrrole-H), 5.63 (t, 2H, J = 7.7 Hz, m- phenylene-H), 2.40 (s, 12H, Me–H), 2.25 (s, 12H, Me–H), 2.18 (s, 12H, Me–H) ppm; 13 C NMR (126 MHz) (CDCl 3 ): δ = 169.2, 152.8, 138.9, 137.7, 137.7, 137.5, 135.8, 134.2, 132.9, 129.5, 128.1, 128.0, 127.3, 126.9, 124.7, 121.0, 21.3, 20.8, and 20.7 ppm; UV/Vis (CH 2 Cl 2 ): λ max ( ε [M –1 cm –1 ]) = 402 (132,023), 551 (48,426), 598 (20,366) nm; HRMS ( m / z ): [M] + calcd. 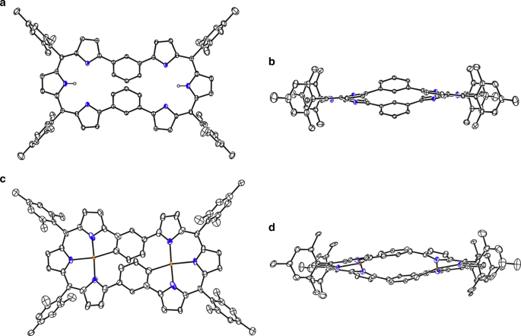Fig. 3: X-ray structures of12and14. aTop view andbside view of12.ctop view, anddside view of14. The thermal ellipsoids are on 30% probability level. Hydrogen atoms except those connected to N atoms are omitted for clarity. Carbon atom, black ellipsoid; nitrogen atom, blue; palladium atom, orange; hydrogen atom small black ball. for C 42 H 36 Br 2 N 5 , 1062.53; found 1062.49. Synthesis of 14 12 (20 mg, 0.019 mmol) was added to a round-bottomed 100 mL flask containing a magnetic bar and dissolved in CHCl 3 /MeOH (15/6 mL). Pd(OAc) 2 (42.6 mg, 0.19 mmol) and NaOAc (18.7 mg, 0.22 mmol) was added, after being refluxed for 24 h, the solvent was evaporated in vacuo. The product was purified by column chromatography on silica-gel (CH 2 Cl 2 /n-hexane as an eluent). Recrystallization with n-hexane gave 14 (17.8 mg, 0.014 mmol, 73.6% yield) as green solids. 1 H NMR (500 MHz) (CDCl 3 ): δ = 8.67 (d, 2H, J = 1.8 Hz, C 6 H 3 -H), 7.59 (d, 2H, J = 4.8 Hz, pyrrole-H), 7.31 (d, 2H, J = 4.7 Hz, pyrrole-H), 7.25 (s, 2H, Ar- m- H), 7.03–7.01 (m, 6H, pyrrole-H and Ar- m- H), 6.98 (s, 2H, Ar- m- H), 6.94 (d, 2H, J = 4.3 Hz, pyrrole-H), 6.67 (d, 2H, J = 4.3 Hz, pyrrole-H), 6.59 (d, 2H, J = 4.3 Hz, pyrrole-H), 5.32 (dd, 2H, J = 7.6, 1.8 Hz, C 6 H 3 -H), 3.95 (d, 2H, J = 7.7 Hz, C 6 H 3 -H), 2.44 (s, 6H, Me–H), 2.41 (s, 6H, Me–H), 2.31 (s, 6H, Me–H), 2.17 (s, 6H, Me–H), 2.16 (s, 6H, Me–H), 2.07 (s, 6H, Me–H); 13 C NMR (126 MHz) (CDCl 3 ): δ = 172.4, 170.7, 170.6, 145.0, 144.2, 144.1, 140.5, 139.4, 139.2, 138.9, 137.8, 137.6, 137.6, 137.5, 137.4, 137.2, 136.7, 135.7, 133.9, 133.2, 132.6, 129.5, 128.0, 127.8, 127.7, 126.3, 126.2, 124.9, 123.7, 119.0, 21.2, 20.8, 20.7, 20.7, and 20.6 ppm; UV/Vis (CH 2 Cl 2 ): λ max ( ε [M –1 cm –1 ]) = 422 (73,384), 599 (17,949), 700 (21,503) nm; HRMS ( m / z ): [M] + calcd. for C 76 H 62 N 6 Pd 2 , 1270.3134; found 1270.3018. Synthesis of 13 Route 1: A p -xylene-DMF solution (3/1.5 mL) of 9 (84.0 mg, 0.12 mmol), 11 (77.7 mg, 0.1 mmol), Pd 2 (dba) 3 (18.5 mg, 0.02 mmol), PPh 3 (21.2 mg, 0.08 mmol), Cs 2 CO 3 (71.0 mg, 0.2 mmol), and CsF (33.4 mg, 0.2 mmol) was degassed through three freeze-pump-thaw cycles, and the reaction Schlenk tube was purged with argon. The resulting mixture was stirred at reflux for 48 h. The reaction mixture was diluted with CHCl 3 , washed with water, and dried over anhydrous sodium sulfate. After the solvent was removed, DDQ (65.8 mg, 0.29 mmol) was added to the resulting mixture in CH 2 Cl 2 stirring for another 8 h. The reaction mixture was passed through a short alumina column (CH 2 Cl 2 as an eluent). Evaporation of the solvent followed by silica-gel column chromatography (CH 2 Cl 2 /n-hexane as an eluent) and recrystallization with CH 2 Cl 2 /MeOH afforded 13 as violet solids (9.6 mg, 0.009 mmol, 9.0% yield). Route 2: A toluene-DMF solution (3/1.5 mL) of 9 (180 mg, 0.25 mmol), 2,6-dibromopyridine (50.0 mg, 0.21 mmol), Pd 2 (dba) 3 (38.8 mg, 0.042 mmol), PPh 3 (44.2 mg, 0.17 mmol), Cs 2 CO 3 (138.0 mg, 0.42 mmol), and CsF (69.5 mg, 0.45 mmol) was degassed through three freeze-pump-thaw cycles, and the reaction Schlenk tube was purged with argon. The resulting mixture was stirred at reflux for 48 h. The reaction mixture was diluted with CHCl 3 , washed with water, and dried over anhydrous sodium sulfate. 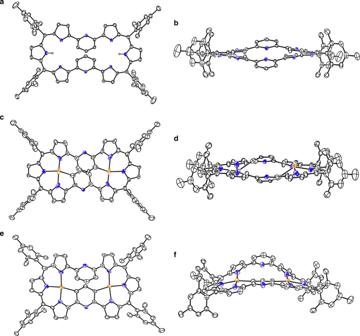Fig. 4: X-ray structures of13,15,and16. aTop view.bSide view of13.cTop view and d) side view of15.eTop view andfside view of16. The thermal ellipsoids are on 30% probability level. Hydrogen atoms are omitted for clarity. Carbon atom, black ellipsoid; nitrogen atom, blue; palladium atom, orange; hydrogen atom small black ball. After the solvent was removed, DDQ (136.2 mg, 0.6 mmol) was added to the resulting mixture in CH 2 Cl 2 and this reaction mixture was stirred for another 8 h. The reaction mixture was passed through a short alumina column (CH 2 Cl 2 as an eluent). Evaporation of the solvent followed by silica-gel column chromatography (CH 2 Cl 2 /n-hexane as an eluent) and recrystallization with CH 2 Cl 2 /MeOH afforded 13 as violet solids (9.1 mg, 0.009 mmol, 8.1% yield). 1 H NMR (500 MHz) (CDCl 3 ): δ = 13.43 (br, 2H, N–H), 7.63 (d, 4H, J = 4.5 Hz, pyrrole-H), 7.41 (d, 4H, J = 8.0 Hz, pyridine-H), 7.01-6.98 (m, 12H, pyrrole-H and Ar- m- H), 6.35 (s, 4H, pyrrole-H), 6.05 (t, 2H, J = 8.0 Hz, pyridine-H), 2.40 (s, 12H, Me–H), 2.26 (s, 12H, Me–H), 2.18 (s, 12H, Me–H) ppm; 13 C NMR (126 MHz) (CDCl 3 ): δ = 169.2, 153.1, 150.8, 139.3, 137.9, 137.6, 137.5, 137.4, 135.2, 134.2, 133.8, 128.2, 128.1, 125.8, 123.5, 121.3, 21.3, 20.8, and 20.7 ppm; UV/Vis (CH 2 Cl 2 ): λ max (ε[M –1 cm –1 ]) = 344 (40,195), 406 (128,444), 555 (46,048), 610 (16,662) nm; HRMS ( m / z ): [M] + calcd. for C 74 H 64 N 8 , 1064.5248; found 1064.5239. Synthesis of 15 , 16 , and 17 13 (19.1 mg, 0.018 mmol) was added to a round-bottomed 100 mL flask containing a magnetic bar, and dissolved in CHCl 3 /MeOH (15/6 mL). Pd(OAc) 2 (40.5 mg, 0.18 mmol) and NaOAc (17.8 mg, 0.21 mmol) was added, after being refluxed for 24 h, the solvent was evaporated in vacuo. 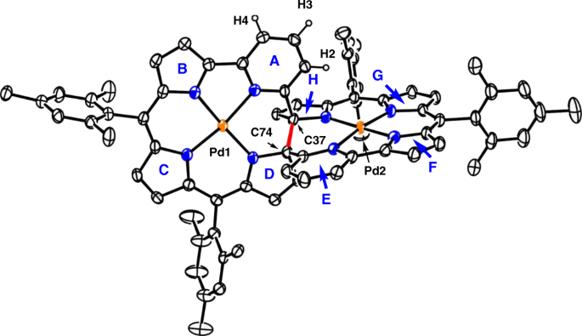Fig. 5: X-ray structure:17. The thermal ellipsoids are on 30% probability level. Hydrogen atoms except those in 2,6-pyridylene are omitted for clarity. Carbon atom, black ellipsoid; nitrogen atom, blue; palladium atom, orange; hydrogen atom small black ball. The residue was purified by column chromatography on silica-gel (CH 2 Cl 2 /n-hexane as an eluent), three fractions were obtained. The first fraction was recrystallized with CH 2 Cl 2 /CH 3 OH to afford 17 (2.8 mg, 2.2 μmol, 12.0% yield) as green solids. 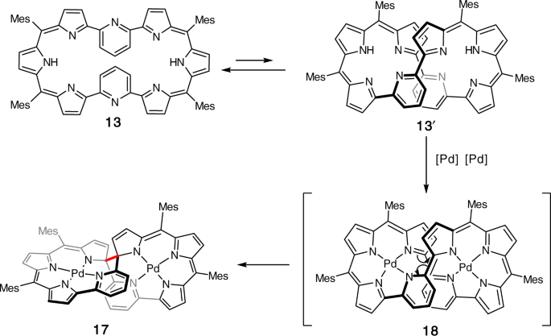Fig. 6: Plausible reaction mechanism from13to17. 13to13′, conformation variation via σ bond rotation;13′to18, metal coordination;18to17, C–C bond (red) forming. 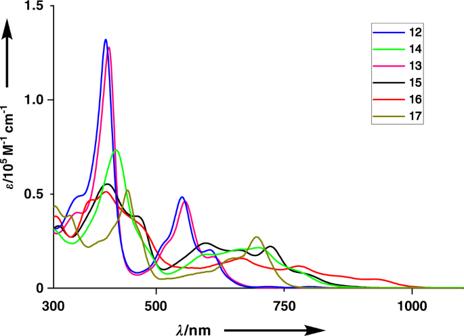Fig. 7: Absorption spectra of12–17in CH2Cl2. UV–Vis–NIR absorption spectra of12(blue), 14 (green),13(purple),15(black),16(red), and17(khaki).λ, wavelength; ε molar extinction coefficient. The second fraction was recrystallized with CH 2 Cl 2 /n-hexane to afford 15 (4.58 mg, 3.6 μmol, 20.0% yield) as dark green solids. The third fraction was recrystallized with CH 2 Cl 2 /CH 3 OH to afford 16 (13.7 mg, 10.8 μmol, 60.0% yield) as navy blue solids. 15: 1 H NMR (500 MHz) (CDCl 3 ): δ = 8.00 (d, 2H, J = 4.7 Hz, pyrrole-H), 7.43 (d, 2H, J = 4.7 Hz, pyrrole-H), 7.34 (d, 2H, J = 4.7 Hz, pyrrole-H), 7.06–7.02 (m, 6H, Ar- m- H), 6.98 (s, 2H, Ar- m- H), 6.94 (d, 2H, J = 4.7 Hz, pyrrole-H), 6.74 (d, 2H, J = 4.5 Hz, pyrrole-H), 6.65 (d, 2H, J = 4.3 Hz, pyrrole-H), 5.46 (d, 2H, J = 7.6 Hz, pyridine-H), 4.07 (d, 2H, J = 7.6 Hz, pyridine-H), 2.44 (s, 6H, Me–H), 2.42 (s, 6H, Me–H), 2.31 (s, 6H, Me–H), 2.18 (s, 6H, Me–H), 2.13 (s, 6H, Me–H), 2.09 (s, 6H, Me–H) ppm; 13 C NMR (126 MHz) (CDCl 3 ): δ = 171.8, 170.7, 162.4, 157.4, 146.2, 144.9, 144.7, 144.1, 141.7, 140.6, 139.6, 138.4, 138.1, 137.7, 137.6, 137.6, 137.3, 136.8, 136.4, 135.5, 134.0, 133.4, 129.2, 128.2, 128.2, 127.0, 125.6, 121.9, 120.5, 21.5, 21.1, 21.0, and 21.0 ppm; UV/Vis (CH 2 Cl 2 ): λ max (ε[M –1 cm –1 ]) = 309 (33,094), 405 (55,309), 461 (38,258), 597 (23,944), 660 (20,273), 723 (22,148) nm; HRMS ( m / z ): [M] + calcd. for C 74 H 60 N 8 Pd 2 , 1272.3038; found 1272.2944. 16: 1 H NMR (500 MHz) (CDCl 3 ): δ = 7.67 (d, 2H, J = 8.0 Hz, pyridine-H), 7.14 (d, 2H, J = 4.5 Hz, pyrrole-H), 7.03 (t, 1H, J = 7.7 Hz, pyridine-H), 6.95–6.92 (m, 12H, Ar- m- H and pyrrole-H), 6.52 (d, 2H, J = 4.9 Hz, pyrrole-H), 6.25 (d, 2H, J = 4.3 Hz, pyrrole-H), 6.22 (d, 2H, J = 4.5 Hz, pyrrole-H), 3.69 (s, 1H, pyridine-H), 2.37 (s, 6H, Me–H), 2.35 (s, 6H, Me–H), 2.21 (s, 6H, Me–H), 2.15 (s, 6H, Me–H), and 2.12 (s, 12H, Me–H) ppm; 13 C NMR (126 MHz) (CDCl 3 ): δ = 175.9, 169.9, 160.9, 155.2, 149.3, 147.4, 146.6, 144.7, 143.0, 140.5, 139.9, 138.0, 137.8, 137.3, 137.2, 137.2, 137.1, 136.8, 135.0, 134.4, 134.2, 133.4, 128.1, 128.0, 127.9, 127.4, 127.0 126.9, 123.2, 121.7, 21.3, 20.8, 20.6, 20.6, and 20.5 ppm; UV/Vis (CH 2 Cl 2 ): λ max (ε[M –1 cm –1 ]) = 403 (51,227), 556 (10,987), 664 (15,863), 777 (11,779), 925 (4759) nm; HRMS ( m / z ): [M] + calcd. for C 74 H 60 N 8 Pd 2 , 1272.3038; found 1272.3063. 17: 1 H NMR (500 MHz) (CDCl 3 ): δ = 7.74 (d, 2H, J = 5.3 Hz, pyrrole-H), 7.44 (t, 2H, J = 7.9 Hz, pyridine-H), 7.31–7.29 (m, 4H, pyridine-H), 6.98–6.93 (m, 10H, Ar- m- H and pyrrole-H), 6.71 (d, 2H, J = 5.0 Hz, pyrrole-H), 6.26–6.24 (m, 4H, pyrrole-H), 6.01 (d, 2H, J = 5.3 Hz, pyrrole-H), 2.38 (s, 6H, Me–H), 2.31 (s, 6H, Me–H), 2.15 (s, 6H, Me–H), 2.09 (s, 6H, Me–H), 2.07 (s, 6H, Me–H), 2.03 (s, 6H, Me–H); 13 C NMR (126 MHz) (CDCl 3 ): δ = 161.2, 157.1, 156.2, 154.7, 147.0, 140.4, 139.9, 139.4, 138.9, 138.0, 137.8, 136.8, 136.7, 134.8, 134.6, 134.5, 133.5, 131.8, 128.1, 128.0, 127.8, 127.7, 125.2, 124.6, 117.0, 116.9, 113.2, 112.1, 100.3, 90.4, 21.2, 21.1, 21.1, 21.0, 20.7, and 20.6 ppm; UV/Vis (CH 2 Cl 2 ): λ max (ε[M –1 cm –1 ]) = 332 (38,615), 444 (51,873), 651 (15,961), 697 (27,095) nm; HR-MS (MALDI-TOF-MS): HRMS ( m / z ): [M] + calcd. for C 74 H 62 N 8 Pd 2 , 1274.3195; found 1274.3141.